Field-induced water electrolysis switches an oxide semiconductor from an insulator to a metal Water is composed of two strong electrochemically active agents, H + and OH − ions, but has not been used as an active electronic material in oxide semiconductors. In this study, we demonstrate that water-infiltrated nanoporous glass electrically switches an oxide semiconductor from insulator to metal. We fabricated a field-effect transistor structure on an oxide semiconductor, SrTiO 3 , using water-infiltrated nanoporous glass—amorphous 12CaO·7Al 2 O 3 —as the gate insulator. Positive gate voltage, electron accumulation, water electrolysis and electrochemical reduction occur successively on the SrTiO 3 surface at room temperature. This leads to the formation of a thin (~3 nm) metal layer with an extremely high electron concentration (10 15 –10 16 cm −2 ), which exhibits exotic thermoelectric behaviour. The electron activity of water as it infiltrates nanoporous glass may find many useful applications in electronics or in energy storage. Water has not been utilized as an active electronic material though water has been widely applied in industry as a coolant (radiators), solvent (batteries) and pressure medium (hydroelectric power generation). We have previously aimed to exploit the electrolysis of water [1] . 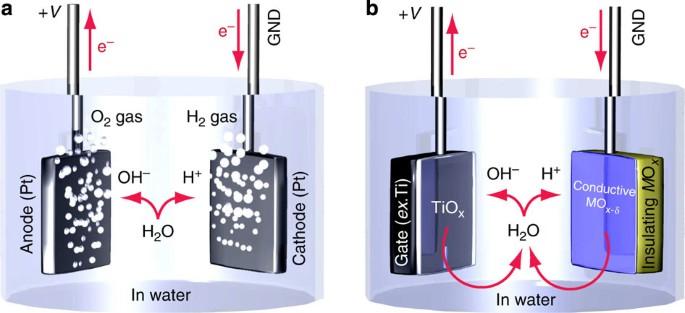Figure 1: Field-induced water electrolysis switches an oxide semiconductor from an insulator to a metal. (a) Simple water electrolysis with two Pt electrodes as the cathode and anode immersed in water. H+and OH−ions, which are generated by the electrolysis, become H2and O2gases on the anode and cathode, respectively. (b) Water electrolysis with an insulating oxideMOx, with a slightly conductive surfaceMOx–δ. Similar toa, H+/OH−ions are attracted to theMOx–−δ, leading to the redox reaction between H+/OH−ions and theMOx–δsurface. GND, ground. Although the electrical conductivity of pure water is extremely low (~0.055 μS cm −1 at 25°C) [2] , ionization of H + and OH − ions occurs when the bias voltage (>1.23 V) is applied between two metallic electrodes immersed in water, as shown in Figure 1a . The ions are then attracted to the cathode and anode. Finally, H 2 and O 2 gases are generated on the cathode and anode, respectively, via the electron transfer on the electrode surface. As H + and OH − ions, which are strong reducing/oxidizing agents for most oxide semiconductors [3] , [4] , [5] , [6] , [7] , [8] , are simultaneously produced in water electrolysis, one may expect that the electrical conductivity of an oxide semiconductor, which is strongly dependent on oxygen non-stoichiometry, can be modulated by utilizing the redox reaction between H + /OH − ions and the oxide surface. However, water electrolysis and the redox reaction do not take place, because no electric field can be applied on the insulating oxide surface in the first place. Thus, the surface of the oxide must be conductive, as schematically shown in Figure 1b . Figure 1: Field-induced water electrolysis switches an oxide semiconductor from an insulator to a metal. ( a ) Simple water electrolysis with two Pt electrodes as the cathode and anode immersed in water. H + and OH − ions, which are generated by the electrolysis, become H 2 and O 2 gases on the anode and cathode, respectively. ( b ) Water electrolysis with an insulating oxide M O x , with a slightly conductive surface M O x–δ . Similar to a , H + /OH − ions are attracted to the M O x–−δ , leading to the redox reaction between H + /OH − ions and the M O x–δ surface. GND, ground. Full size image We have found that water-infiltrated nanoporous glass overcomes this problem and switches an oxide semiconductor from an insulator to a metal. Electron accumulation, water electrolysis and redox take place successively on an oxide surface at room temperature (RT), leading to the formation of a thin metal layer on the oxide. We have fabricated a field-effect transistor (FET) structure with source, drain and gate electrodes on an insulating oxide, using water-infiltrated nanoporous glass as the gate insulator. First, the insulating oxide surface becomes slightly conductive by applying the gate voltage because of electrostatic charge accumulation. Then, water electrolysis occurs between the gate and the oxide surface. Finally, a redox reaction takes place between H + /OH − ions and the oxide surface. As a result, a thin metal layer is formed on an insulating oxide. The key material to make the best use of the electron activity of water is nanoporous glass. We chose amorphous 12CaO·7Al 2 O 3 ( a -C12A7) with a nanoporous structure for this purpose. C12A7 is an abundant and environmentally benign material. Crystalline C12A7 becomes semiconducting [9] or metallic [10] , [11] when the clathrated free oxygen ions (O 2− ), which are incorporated into the cage structure (~0.4 nm in diameter), are removed by chemical reduction treatment. On the other hand, 'amorphous' C12A7 is a good electrical insulator, because amorphous C12A7 does not have a cage structure, we therefore ruled out the possibility of electrical conductivity of an amorphous C12A7 film. As C12A7 can be hydrated easily [12] , it is used commercially as a major constituent of aluminous cement. In 1987, Hosono and Abe [13] found that a large amount of bubbles was generated in an a -C12A7 glass, when C12A7 melt was quenched under high oxygen pressure. In the present study, we develop a method to fabricate a -C12A7 film with nanoporous structure (CAN, hereafter) by pulsed laser deposition. In this study, we show that water-infiltrated CAN electrically switches an oxide semiconductor from insulator to metal, using a CAN-gated FET structure on a SrTiO 3 single crystal ( Fig. 2a ) as a proof of concept. Although SrTiO 3 is a wide bandgap (~3.2 eV) insulator, it becomes n -type conducting SrTiO 3 −δ by appropriate reducing treatments [5] . Conducting SrTiO 3 , especially when it is a two-dimensional (2D) conductor [14] , [15] , is of great importance as an active material for future electronic devices [16] , because it has several potential advantages over conventional semiconductor-based electronic materials, such as transparency [17] , giant magnetoresistance [18] and giant thermopower [19] . On applying positive gate voltage to the CAN-gated SrTiO 3 FET, electron accumulation, water electrolysis and electrochemical reduction occur successively on the SrTiO 3 surface at RT. This leads to the formation of a thin (~3 nm) metal layer with an extremely high electron concentration (10 15 –10 16 cm −2 ), which exhibits exotic thermoelectric behaviour. 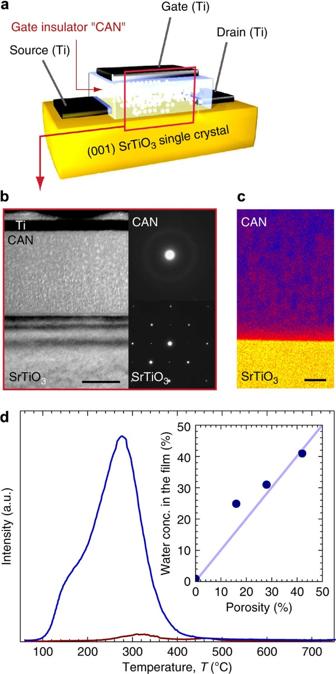Figure 2: The CAN-gated SrTiO3FET. (a) A schematic illustration of the CAN-gated SrTiO3FET. (b) Cross-sectional TEM image of the CAN-gated SrTiO3FET (left panel). Scale bar is 100 nm. Trilayer structure composed of Ti/CAN/SrTiO3is observed. Large amount of light spots are seen in the whole CAN region. Broad halo is observed in the selected area electron diffraction pattern of CAN, and diffraction pattern from SrTiO3single crystal is also shown below (right panel). (c) Z-contrast, high-angle, annular dark-field STEM image of the CAN/SrTiO3interface. Scale bar is 20 nm. Nanopores with diameter <10 nm appear dark. (d) TDS spectrum of water (m/z=18 H2O) in the CAN film (blue). The amount of H2O up to 400°C was estimated to be 1.4×1022cm−3(=0.41 g cm−3, ~41%). TDS spectrum in the densea-C12A7 film is shown for comparison (red, 0.009 g cm−3). The water concentration increases monotonically with an increase in the porosity of the CAN films (the inset). Figure 2: The CAN-gated SrTiO 3 FET. ( a ) A schematic illustration of the CAN-gated SrTiO 3 FET. ( b ) Cross-sectional TEM image of the CAN-gated SrTiO 3 FET (left panel). Scale bar is 100 nm. Trilayer structure composed of Ti/CAN/SrTiO 3 is observed. Large amount of light spots are seen in the whole CAN region. Broad halo is observed in the selected area electron diffraction pattern of CAN, and diffraction pattern from SrTiO 3 single crystal is also shown below (right panel). ( c ) Z-contrast, high-angle, annular dark-field STEM image of the CAN/SrTiO 3 interface. Scale bar is 20 nm. Nanopores with diameter <10 nm appear dark. ( d ) TDS spectrum of water ( m / z =18 H 2 O) in the CAN film (blue). The amount of H 2 O up to 400°C was estimated to be 1.4×10 22 cm −3 (=0.41 g cm −3 , ~41%). TDS spectrum in the dense a -C12A7 film is shown for comparison (red, 0.009 g cm −3 ). The water concentration increases monotonically with an increase in the porosity of the CAN films (the inset). Full size image Water-infiltrated nanoporous glass (CAN) The trilayer structure composed of Ti (20 nm)/CAN (200 nm)/SrTiO 3 is clearly observed in the cross-sectional transmission electron microscopic (TEM) image of the CAN-gated SrTiO 3 FET ( Fig. 2b ). Many brighter contrasts (diameter ~10 nm) are seen throughout the CAN region. Furthermore, several dark contrasts with a diameter <10 nm are observed in the Z-contrast, high-angle, annular dark-field scanning TEM (STEM) image of the CAN film ( Fig. 2c ). Judging from these TEM/STEM images, high-density nanopores with a diameter of <10 nm are incorporated into the CAN film. We subsequently measured thermal desorption spectrum (TDS) of the CAN films to detect weakly bonded chemical species in the nanopores. Most of the desorbed species were H 2 O ( m / z =18, where m / z indicates the molecular mass to charge ratio; Fig. 2d ). The amount of H 2 O up to 400°C was estimated to be 1.4×10 22 cm −3 , which corresponds to 41%. The bulk density of the CAN film was ~2.1 g cm 3 , evaluated by grazing incidence X-ray reflectivity ( Supplementary Fig. S2 ), which corresponds to 72% of fully dense a -C12A7 (2.92 g cm 3 ) [20] . From these results, we judged that moisture in the air (humidity 40–50%) would infiltrate the CAN film most likely due to the capillary effect, hence, nanopores in the CAN film were filled with water. Field-induced water electrolysis We then measured the electron transport properties of the CAN-gated SrTiO 3 FET at RT. 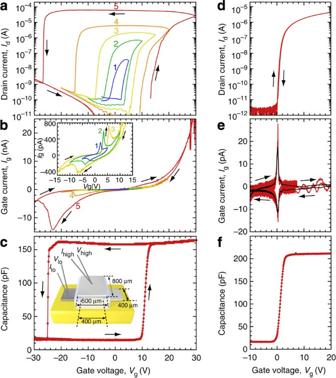Figure 3: Electron transport properties of the CAN-gated SrTiO3FET at RT. (a)IdversusVg, (b)IgversusVgand (c)CversusVg,IdversusVg(d),IgversusVg(e), andCversusVgcurves (f) of the densea-C12A7-gated SrTiO3FET are also shown for comparison. Both the channel length,L, and the channel width,W, are 400 μm. The gate voltage sweeps were performed in numerical order (for example: 1: −5 V→0 V→+5 V→0 V→–5 V). (a)IdversusVgcurves (Vd=+2 V) show large anticlockwise hysteresis, although very small clockwise hysteresis is seen in the dense one (d,Vd=+1 V). (b)Igincreases exponentially up to 20 nA withVg, which is ~104greater than that of the densea-C12A7-gated SrTiO3FET (e, red: observed, grey: smoothed). (c) TheCversusVgcurve shows a large anticlockwise hysteresis loop. The maximumC(frequency: 20 Hz) of the nanoporousa-C12A7-gated SrTiO3FET is ~160 pF, ~76% of that of the densea-C12A7-gated SrTiO3FET ((f) ~210 pF). Figure 3 summarizes (a) drain current ( I d ) versus gate voltage ( V g ) curves, (b) gate current ( I g ) versus V g curves, and (c) capacitance ( C ) versus V g curve of the CAN-gated SrTiO 3 FET. Corresponding properties of the dense a -C12A7-gated SrTiO 3 FET [21] (d, e, f) were also measured for comparison. Both the channel length, L , and the channel width, W , were 400 μm. Dielectric permittivity ( ϵ r ) of a -C12A7 was 12 [21] . The gate voltage sweeps were performed in numerical order (for example: 1:−5 V→0 V→+5 V→0 V→–5 V). The I d versus V g curves (a) show large anticlockwise hysteresis, indicating movement of mobile ions [22] , though very small clockwise hysteresis (~0.5 V) is seen in the dense a -C12A7-gated SrTiO 3 FET (d). Although very small, I g (~2 pA) is observed in the dense a -C12A7-gated SrTiO 3 FET (e), whereas the I g of the CAN-gated SrTiO 3 FET (b) increases exponentially up to 20 nA with V g , suggesting that mobile ions transport electronic charge. The C versus V g curve (c) of the CAN-gated SrTiO 3 FET shows large anticlockwise hysteresis loop. The maximum C is ~160 pF, ~76% of the value for the dense a -C12A7-gated SrTiO 3 FET ((f) ~210 pF), consistent with the fact that the volume fraction of dense a -C12A7 part in the CAN film is ~72%. Figure 3: Electron transport properties of the CAN-gated SrTiO 3 FET at RT. ( a ) I d versus V g , ( b ) I g versus V g and ( c ) C versus V g , I d versus V g ( d ), I g versus V g ( e ), and C versus V g curves ( f ) of the dense a -C12A7-gated SrTiO 3 FET are also shown for comparison. Both the channel length, L , and the channel width, W , are 400 μm. The gate voltage sweeps were performed in numerical order (for example: 1: −5 V→0 V→+5 V→0 V→–5 V). ( a ) I d versus V g curves ( V d =+2 V) show large anticlockwise hysteresis, although very small clockwise hysteresis is seen in the dense one ( d , V d =+1 V). ( b ) I g increases exponentially up to 20 nA with V g , which is ~10 4 greater than that of the dense a -C12A7-gated SrTiO 3 FET ( e , red: observed, grey: smoothed). ( c ) The C versus V g curve shows a large anticlockwise hysteresis loop. The maximum C (frequency: 20 Hz) of the nanoporous a -C12A7-gated SrTiO 3 FET is ~160 pF, ~76% of that of the dense a -C12A7-gated SrTiO 3 FET (( f ) ~210 pF). Full size image We also observed a clear pinch-off and saturation in I d at low V g region (see Supplementary Fig. S3 ), indicating that the operation of this FET conformed to standard FET theory at low gate voltage. Thus, we concluded that first the insulating SrTiO 3 surface became slightly conductive with gate voltage because of the electron charge that was accumulated at the SrTiO 3 surface by pure electrostatic effect. To clarify the role of water in the electrical transport properties, we measured the I d versus V g characteristics of the CAN-gated SrTiO 3 FET at 0°C using a Peltier cooler, because H + and OH+− ions cannot move through ice ( Supplementary Fig. S4 ). The device does not show such large anticlockwise hysteresis at 0°C. Although the maximum C increased from ~160 pF (25°C) to ~240 pF (0°C), I d at V g =+10 V decreased from ~5 μA (25°C) to ~1 μA (0°C), most likely because of the fact that water in the CAN acts as a simple gate dielectric at 0°C ( ϵ r 25°C ~78, ϵ r 0°C ~88) [23] . The field-effect mobility ( μ FE ) value of the FET at 0°C is ~0.8 cm 2 V −1 s −1 , which is comparable to that of the dense a -C12A7-gated SrTiO 3 FET (~2 cm 2 V −1 s −1 ), obtained from μ FE = g m (( C × V d )/( W × L )) −1 , where g m was the transconductance ∂ I d /∂ V g . We also measured Hall mobility ( μ Hall ) of a CAN-gated SrTiO 3 FET after several V g applications (metallic state) and obtained μ Hall values of 2.3–2.5 cm 2 V −1 s −1 , which is approximately three times larger than the ì FE value (~0.8 cm 2 V −1 s −1 ). These results clearly indicate that H + and OH+− ions in the CAN are the main contributors to electron transport at RT. Insulator-to-metal switching We then observed the electrochemical redox reaction of SrTiO 3 . 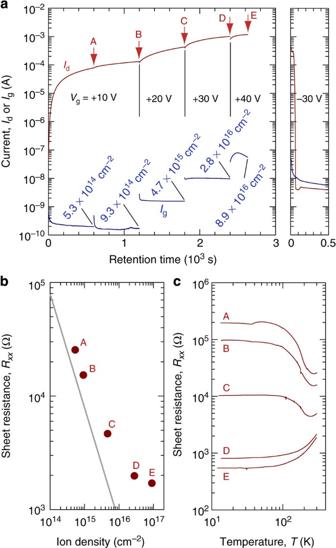Figure 4: A redox reaction switches an insulating SrTiO3to metal. (a) Retention time dependences ofIdandIgfor the CAN-gated SrTiO3FET at severalVgat RT (Vd=+2 V). TheIdincreases gradually with retention time at constantVg. Ion density, which is the retention time integral ofIg, reaches ~9×1016cm−2whenVg=+40 V is applied. (b)Rxxversus ion density for the state A–E marked inaat RT. The grey line (slope=–1) indicatesRxx=(e·nxx·μ)−1, wherenxxandμare ion density, andμFE(0.8 cm2V−1s−1), which was obtained as in SupplementaryFigure S4b. (c) Temperature dependence ofRxxfor the state A–E marked inFigure 4a. Figure 4a shows the changes of I d and I g during V g sweep from +10 to +40 V, as a function of retention time. The I d gradually increases with retention time. The rate of I d increase grows with V g . The I g also increases with V g . The I d reaches ~1 mA at V g =+40 V. The I d decreases drastically when negative V g of −30 V is applied. Figure 4: A redox reaction switches an insulating SrTiO 3 to metal. ( a ) Retention time dependences of I d and I g for the CAN-gated SrTiO 3 FET at several V g at RT ( V d =+2 V). The I d increases gradually with retention time at constant V g . Ion density, which is the retention time integral of I g , reaches ~9×10 16 cm −2 when V g =+40 V is applied. ( b ) R xx versus ion density for the state A–E marked in a at RT. The grey line (slope=–1) indicates R xx =( e · n xx · μ ) −1 , where n xx and μ are ion density, and μ FE (0.8 cm 2 V −1 s −1 ), which was obtained as in Supplementary Figure S4b . ( c ) Temperature dependence of R xx for the state A–E marked in Figure 4a . Full size image The sheet resistance ( R xx ) at several points (A–E) was plotted as a function of ion density, which was obtained by I g × t ( Fig. 4b ). The observed values were close to the grey line, which is R xx =( e · n xx · μ ) −1 , where n xx and μ are ion density, and μ FE (0.8 cm 2 V −1 s −1 ) was obtained as in Supplementary Figure S4b , suggesting that carrier electrons were generated as a result of the electrochemical reduction of SrTiO 3 . Although samples A–C exhibit insulating R xx − T behaviour, D and E exhibit metallic R xx − T behaviour ( Fig. 4c ). Exotic thermopower We have also shown that the metal layer on the SrTiO 3 in the FET exhibits novel thermoelectric behaviour: V-shaped turnaround of S is seen, although R xx decreases gradually as V g increases ( Fig. 5 ). As we have reported previously, | S | value enhancement of electron-doped SrTiO 3 can be observed when the conducting layer thickness is <~3 nm [19] , probably because of 2D effect [24] , where the thermal de Broglie's wavelength of conduction electrons in SrTiO 3 is ~6 nm [25] . We therefore expected that 2D | S | can be observed at high V g , because the layer thickness may become thinner. 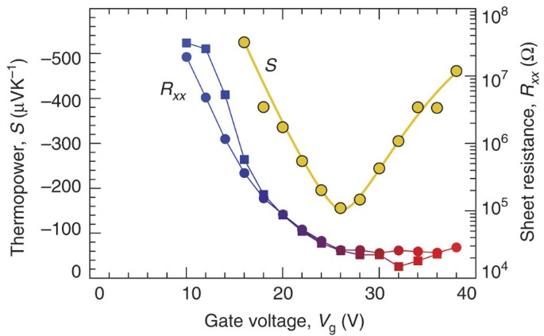Figure 5: Thermopower and sheet resistance as a function of appliedVg. Novel thermopower behaviour: V-shaped turnaround ofSis seen, thoughRxx(circle: beforeSmeasurement, square: afterSmeasurement) decreases gradually asVgincreases, probably due to transition of electronic nature from 3D to 2D in the interface region. Figure 5: Thermopower and sheet resistance as a function of applied V g . Novel thermopower behaviour: V-shaped turnaround of S is seen, though R xx (circle: before S measurement, square: after S measurement) decreases gradually as V g increases, probably due to transition of electronic nature from 3D to 2D in the interface region. Full size image When the V g was <+26 V, | S | value gradually decreased with V g . Similar | S | behaviour, which can be analysed using simple three-dimensional (3D) electron diffusion theory, was also observed in the dense a -C12A7-gated SrTiO 3 FET, as shown in Supplementary Figure S5 . Thus, we used the 3D electron diffusion theory [26] to analyse the layer thickness. The 3D electron concentrations ( n 3D ) at V g =+16, +20 and +26 V were estimated to be ~1.5×10 19 , 1.5×10 20 and ~1.1×10 21 cm −3 , respectively. The n xx values at V g =+16, +20 and +26 V, which can be calculated using R xx and μ FE (0.8 cm 2 V −1 s −1 ), are 1.4×10 13 , 9.0×10 13 and 3.3×10 14 cm −2 , respectively, suggesting that the SrTiO 3– δ thicknesses (~ n xx / n 3D ) are ~9, 6 and 3 nm, respectively, confirming that the observed S obeys simple 3D electron diffusion theory. On the contrary, when the V g >26 V was applied, the | S | value increased. The conducting layer thickness may be <3 nm, the observed upturn at V g >26 V is most likely due to 2D effect [19] , [24] . The present CAN-gated SrTiO 3 FET has several merits compared with established methods such as thermal reduction [5] , ion irradiation [17] , [27] , thin film growth [14] , [15] , [17] , [18] and simple FET [21] , [28] , which are often utilized to switch an insulating SrTiO 3 to a metal. This is because the current method allows a metal layer to be easily fabricated with extremely low energy. First, required electricity is extremely less (~50 μW cm −2 for 'D' in Fig. 4 ) compared with that of thermal reduction (~kW) and ion implantation (~W cm −2 ). Second, an extremely thin (~3 nm) metal layer, which exhibits exotic thermopower ( Fig. 5 ), can be fabricated. Normally, such thin layers must be fabricated through complicated vapour phase epitaxy methods, such as pulsed laser deposition and molecular beam epitaxy. Third, our CAN-gated SrTiO 3 FET exhibits a nonvolatile metal or highly conductive/insulator transition ( Figs 3a and 4a and Supplementary Fig. S6 ), because a reversible redox reaction is utilized in addition to the field effect. Although several efficient gating methods using liquid electrolytes have been proposed very recently [28] , [29] , [30] , [31] , we would like to argue that the present water-infiltrated nanoporous glass 'CAN' is truly superior to the liquid-based gate dielectrics. Liquid electrolytes including 'gel' would be very useful to electrostatically accumulate carriers at the transistor channel by applying rather low V g (a few volts) using their huge capacitance. However, they would not be suitable for practical applications without sealing because of liquid leakage problem. Our 'CAN' is a chemically stable rigid glassy solid with a higher decomposition voltage, showing excellent adhesion with chemically robust oxide such as SrTiO 3 surface and no liquid (water) leakage occurs. Carrier injection/discharge can be controlled by V g as redox reaction, which occurs at the interface of H + or OH − /semiconductor, is utilized for carrier injection/discharge, though rather high V g (several ten volts) should be required for Redox reaction. Further, we observed novel thermopower behaviour: V-shaped turnaround, probably due to transition of electronic nature from 3D to 2D in the interface region, as the FET could be operated at high V g . These clearly indicate the effectiveness of our 'CAN'. In summary, we have demonstrated that water, when it infiltrates nanoporous glass, can switch an insulating oxide to metal. As an example, we have built a FET on an insulating oxide, SrTiO 3 , using water-infiltrated nanoporous glass, amorphous 12CaO·7Al 2 O 3 with nanoporous structure 'CAN' as the gate insulator. First, the insulating SrTiO 3 surface became slightly conductive with gate voltage because of electrostatic charge accumulation. Then, H + /OH − ions were generated due to water electrolysis occurring between the gate and the SrTiO 3 surface. Subsequently, a redox reaction took place between H + /OH − ions and the SrTiO 3 surface. As a result, a thin metal (~3 nm) layer with extremely high electron concentration of 10 15 –10 16 cm −2 was formed on the insulating SrTiO 3 . The electron activity of water, as it infiltrates nanoporous glass 'CAN', may find many useful applications in electronics or energy storage. Fabrication of the CAN-gated SrTiO 3 FET The FET structures ( Fig. 2a ) were fabricated on the (001)-face of SrTiO 3 single crystal plate (10×10×0.5 mm, SHINKOSHA), treated in NH 4 F-buffered HF (BHF) solution [32] . First, 20-nm-thick metallic Ti films, used as the source and drain electrodes, were deposited through a stencil mask by electron beam evaporation (base pressure ~10 4 Pa, no substrate heating/cooling) onto the SrTiO 3 plate. Ohmic contact between the Ti and SrTiO 3 surface was confirmed by conventional I – V characteristics (output characteristics), as shown in Supplementary Figure S3b . Then, a 200-nm-thick CAN film was deposited through a stencil mask by pulsed laser deposition (KrF excimer laser, fluence ~3 J cm 2 per pulse) at RT using dense polycrystalline C12A7 ceramic as target. During the CAN deposition, the oxygen pressure in the deposition chamber was kept at 5 Pa. Finally, a 20-nm-thick metallic Ti film, used as the gate electrode, was deposited through a stencil mask by electron beam evaporation. Analysis of the CAN films The bulk density and thickness of the CAN films were evaluated by grazing incidence X-ray reflectivity (ATX-G, Rigaku). Microstructures of the CAN films were observed by using TEM (JEOL JEM-2010, acceleration voltage=200 kV) and aberration-corrected STEM (JEOL JEM-2100F, acceleration voltage=200 kV). Water concentration in the CAN films was analysed by TDS measurements (TDS1200, ESCO). The TDS measurements were carried out in a vacuum chamber with the background pressure of ~10 −7 Pa at varied temperatures from 60 to 700°C at a heating rate of 60°C per min. Electron transport properties Electrical properties of the FETs were measured by using a semiconductor device analyser (B1500A, Agilent). The capacitance of the CAN layer on the FETs was measured using an LCR meter (4284A, Agilent). The thermopower ( S ) values were measured using two Peltier devices under the FET to give a temperature difference between the source and drain electrodes ( Supplementary Fig. S7 ). Two thermocouples (K-type) located at both ends of the channel were used for monitoring the temperature difference (Δ T , 0–5 K). S values were measured after each V g sweep (for example: V g application 0 V→+16 V→0 V→ S measurements). How to cite this article: Ohta, H. et al . Field-induced water electrolysis switches an oxide semiconductor from an insulator to a metal. Nat. Commun. 1:118 doi: 10.1038/ncomms1112 (2010).